Self-recognition of the endothelium enables regulatory T-cell trafficking and defines the kinetics of immune regulation Localization of CD4 + CD25 + Foxp3 + regulatory T (Treg) cells to lymphoid and non-lymphoid tissue is instrumental for the effective control of immune responses. Compared with conventional T cells, Treg cells constitute a minute fraction of the T-cell repertoire. Despite this numeric disadvantage, Tregs efficiently migrate to sites of immune responses reaching an optimal number for the regulation of T effector (Teff) cells. The array and levels of adhesion and chemokine receptor expression by Tregs do not explain their powerful migratory capacity. Here we show that recognition of self-antigens expressed by endothelial cells in target tissue is instrumental for efficient Treg recruitment in vivo . This event relies upon IFN-γ-mediated induction of MHC-class-II molecule expression by the endothelium and requires optimal PI3K p110δ activation by the T-cell receptor. We also show that, once in the tissue, Tregs inhibit Teff recruitment, further enabling a Teff:Treg ratio optimal for regulation. Naturally occurring regulatory T cells (Treg), defined as CD4 + CD25 + Foxp3 + T cells, play a non-redundant role in the maintenance of physiological tolerance to self-antigens and prevention of autoimmune responses [1] , [2] . Treg generation in the thymus is promoted by the recognition of self-peptides with intermediate affinity [3] . Recognition of self-antigen is also required for mature Tregs activation and function [4] . Tregs exert their immunomodulatory role both in lymphoid and non-lymphoid tissue. Localization of Tregs in the lymph nodes (LNs) is instrumental for the regulation of T-cell expansion and differentiation [5] , however, once the effector response is established, regulation of local inflammation in target tissue becomes crucial [6] , [7] . Several studies in autoimmunity have highlighted the importance of the co-localization of Tregs with effector T cells (Teff) in non-lymphoid target tissues. For example, in Foxp3-deficient Scurfy mice, widespread autoimmune disease develops that may be prevented by treatment with Tregs. However, restoration of the Treg compartment with a-1,3-fucosyltransferase VII-deficient Tregs that are incapable of migrating to skin results in the prevention of autoimmune disease in all tissues but the skin [8] . Similarly, the loss of CCR4 expression in Tregs prevents their migration to both the skin and lungs, resulting in skin and lung inflammatory disease [9] . An optimal Treg:Teff ratio, in which over 30% of the infiltrating T cells are Tregs, is necessary to achieve regulation in non-lymphoid tissue [10] . To reach this proportion, rapid accumulation of Treg relative to Teff infiltration is required to control tissue damage [11] , further emphasizing the importance of effective Treg recruitment. The minute proportion of Tregs in the peripheral blood (2–5%) and their poor proliferative capacity suggest that mechanisms must be in place which favour their convergence and localization to the inflammatory site. Like Teff cells, activated Tregs also utilize distinct chemokine receptor and integrin expression to support their trafficking and retention at sites where regulation is required [12] , [13] , [14] . For example, activated Tregs express α E β 7 , which binds its ligand E-cadherin and allows efficient localization into inflamed tissue to suppress the effector phase of immune response [15] , [16] . However, these molecular interactions do not fully account for the powerful migratory activity of Tregs and their rapid access to and accumulation in non-lymphoid tissue relative to Teff. Importantly, Treg-mediated suppression must be coordinated with that of effector responses so that the regulatory phase develops with a sufficient delay to allow the effector phase to ensue, but prior to the occurrence of tissue damage [11] . The mechanism coordinating these migratory events is not known. There is evidence that Treg trafficking requires antigen recognition. A recent study has suggested that compartmentalization of Treg cells within LNs may be governed by antigen recognition as indicated by the enrichment of recently activated, CD69-expressing Tregs in LNs following adoptive transfer [17] . Similarly, mice expressing a Ox40-cre allele that is prominently expressed in Treg cells, and a conditional null allele of the gene encoding p56Lck, displayed abnormal Treg homeostasis characterized by preferential redistribution to the LNs, but not to non-lymphoid tissue [18] . Given the well-established specificity of Tregs for self-derived peptides, we tested the hypothesis that antigen recognition promotes the rapid recruitment of Tregs to inflamed tissue to reach functionally regulatory numbers. Here we show that self-antigen presentation by the endothelium leads to efficient Treg migration into target tissue in vivo . IFN-γ-mediated induction of MHC-class-II molecule expression by the endothelium is critical to this event. We further show that, once localized in the tissue, Tregs inhibit Teff recruitment, thus favouring the establishment of a Teff:Treg ratio which allows functional regulation. On the basis of the findings described here, we propose that recognition of antigen displayed by inflamed vascular endothelium is required for the efficient and coordinated recruitment of Treg cells to target tissue and defines the kinetics of Treg-mediated regulation. Self-recognition is required for Treg trafficking To establish whether self-recognition regulates naturally occurring Treg cell (Tregs) trafficking to non-lymphoid tissue in physiological settings, we adapted a well-established model of T-cell recruitment to antigen-enriched peritoneum. In this model, local presentation of endogenous peptides is achieved by intraperitoneal (i.p.) administration of a low dose of IFN-γ, which induces local upregulation of MHC molecules [19] . We first compared the recruitment of Tregs from the circulation into the peritoneum of syngeneic (C57BL/6, H2 b ) and irrelevant (CBA/CA, H2 k ) mice. To minimize the effects of in vitro manipulation, CD4 + T cells isolated by immunomagnetic negative selection from Foxp3-GFP reporter mice [20] (10 7 /mouse) were pooled (to ensure that the same number of Tregs in the cell preparation) and injected intravenously (i.v.) in IFN-γ-treated or untreated recipients. As it is shown in Fig. 1a,b , significantly larger numbers of green fluorescent protein (GFP)-tagged Tregs migrated to the peritoneal cavity of syngeneic recipients previously exposed to IFN-γ, compared with those detected in the lavage of IFN-γ-treated irrelevant (CBA/Ca) mice and non-treated syngeneic recipients. Notably, 50% of the Tregs recruited in the peritoneal cavity and draining LNs (dLNs) upregulated CD69 expression, indicative of recent T-cell receptor (TCR) engagement in this cell population ( Fig. 1c ). Similar observations were made when irrelevant BALB/c (H2 d ) recipients were used ( Supplementary Fig. 1 ). Treg cells also preferentially accumulated in (mesenteric) dLNs of IFN-γ-treated syngeneic, but not irrelevant mice, suggesting that antigen presentation also affects their localization to secondary lymphoid tissue, as previously suggested [17] . 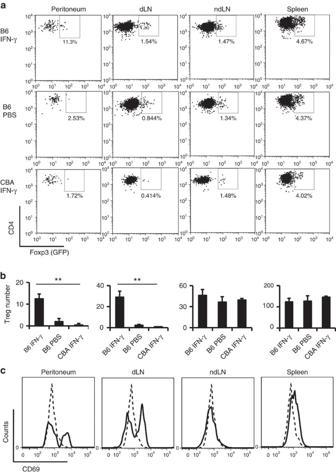Figure 1: Antigen recognition facilitates Treg trafficking. Total CD4+ T cells from FoxP3-eGFP reporter mice (107/mouse) were injected intravenously into syngeneic C57BL/6 or irrelevant CBA (H2k) mice that had received an intraperitoneal injection of 600 U IFN-γ 72 h earlier. Some C57BL/6 recipient received saline solution alone. The presence of GFP+Tregs in lavage, dLN and spleen was analysed by flow cytometry 16 h later. Tregs were identified by gating on the CD4+GFP+population. Representative dot plots are shown in panela. The mean number of Treg cells (in the total CD4+population) of Treg cells detected in the peritoneal cavity and lymphoid organs is shown in panelb. Error bars represent s.d. Statistical significance was calculated with unpaired Student’st-test. (n=3,N=4) **P<0.01. (c) GFP+Tregs retrieved in the same sites from IFN-γ-treated syngeneic C57BL/6 recipients were stained with anti-CD69-PE/Cy7 (clone H1.2F3). CD69 expression was analysed by flow cytometry. The dotted line shows non-specific staining with an Isotype-matched control antibody. The histograms are representative of three cell preparations. Figure 1: Antigen recognition facilitates Treg trafficking. Total CD4+ T cells from FoxP3-eGFP reporter mice (10 7 /mouse) were injected intravenously into syngeneic C57BL/6 or irrelevant CBA (H2 k ) mice that had received an intraperitoneal injection of 600 U IFN-γ 72 h earlier. Some C57BL/6 recipient received saline solution alone. The presence of GFP + Tregs in lavage, dLN and spleen was analysed by flow cytometry 16 h later. Tregs were identified by gating on the CD4 + GFP + population. Representative dot plots are shown in panel a . The mean number of Treg cells (in the total CD4 + population) of Treg cells detected in the peritoneal cavity and lymphoid organs is shown in panel b . Error bars represent s.d. Statistical significance was calculated with unpaired Student’s t- test. ( n =3, N =4) ** P <0.01. ( c ) GFP + Tregs retrieved in the same sites from IFN-γ-treated syngeneic C57BL/6 recipients were stained with anti-CD69-PE/Cy7 (clone H1.2F3). CD69 expression was analysed by flow cytometry. The dotted line shows non-specific staining with an Isotype-matched control antibody. The histograms are representative of three cell preparations. Full size image To further confirm that Treg localization is driven by antigen recognition, we tested the possibility that, within a polyclonal Treg population, Tregs are selectively recruited based on their TCR specificity. To this aim, we enriched GFP-tagged Tregs cross-reactive for H2 d alloantigens by in vitro culture with BALB/c-derived immature dendritic cells (DCs) and IL-2 (ref. 21 ). In vitro culture did not affect Treg phenotype and regulatory activity, which however shifted towards the alloantigen with time ( Fig. 2a–c ). We then compared the recruitment of circulating allospecific Tregs into the peritoneum of IFN-γ-treated (i.p.) allogeneic BALB/c, syngeneic C57BL/6 and irrelevant CBA recipients. As shown in Fig. 2d,e , allospecific Tregs migrated more efficiently to the peritoneal cavity of allogeneic BALB/c mice compared with that of syngeneic C57BL/6 and irrelevant CBA mice. Similar to what we observed in the experiments with freshly isolated Tregs, this effect was accompanied by enhanced allospecific Treg recruitment in the dLNs of IFN-γ-treated alloantigen-expressing recipients. 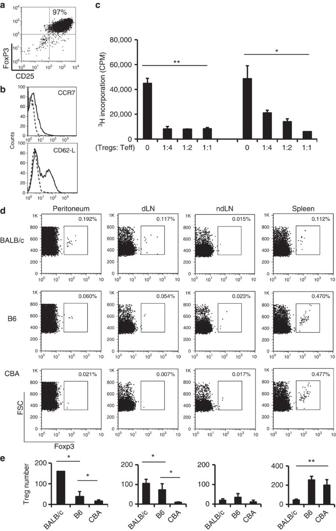Figure 2: Allospecific Tregs migrate more efficiently to the peritoneal cavity of allogeneic mice. Allospecific Tregs (H2b) were expanded byin vitroculture with BALB/c-derived, (H2d) immature DCs and IL-2. Key phenotypic markers are depicted in panelsa(CD25 and FoxP3) andb(CCR7 and CD62L). In panelc, increasing numbers of allospecific Tregs were added to co-cultures of C57BL/6 conventional naïve T cells (105) stimulated with BALB/c-derived DCs (103), or CD3/CD28 beads. T-cell proliferation was measured as3HTdR incorporation in triplicate cultures (N=5). Error bars represent s.d. Statistical significance was calculated with unpaired Student’st-test. *P<0.05, **P<0.01. Panelsd,e: CFSE-labelled H2d-allospecific Treg cells were injected intravenously (107/mouse) into alloantigenic BALB/c, syngeneic C57BL/6 or irrelevant CBA (H2k) mice that had received an intraperitoneal injection of 600 U IFN-γ 72 h earlier. The presence of GFP+Tregs in lavage, mesenteric dLNs, non-dLNs and spleen was analysed by flow cytometry 16 h later. Representative dot plots are shown in paneld. The mean number of Treg cells (in the total CD4+population) detected in the peritoneal cavity and lymphoid organs is shown in panele. Error bars represent s.d. Statistical significance was calculated with unpaired Student’st-test. (n=3,N=4) *P<0.05, **P<0.01. Figure 2: Allospecific Tregs migrate more efficiently to the peritoneal cavity of allogeneic mice. Allospecific Tregs (H2 b ) were expanded by in vitro culture with BALB/c-derived, (H2 d ) immature DCs and IL-2. Key phenotypic markers are depicted in panels a (CD25 and FoxP3) and b (CCR7 and CD62L). In panel c , increasing numbers of allospecific Tregs were added to co-cultures of C57BL/6 conventional naïve T cells (10 5 ) stimulated with BALB/c-derived DCs (10 3 ), or CD3/CD28 beads. T-cell proliferation was measured as 3 HTdR incorporation in triplicate cultures ( N =5). Error bars represent s.d. Statistical significance was calculated with unpaired Student’s t -test. * P <0.05, ** P <0.01. Panels d , e : CFSE-labelled H2 d -allospecific Treg cells were injected intravenously (10 7 /mouse) into alloantigenic BALB/c, syngeneic C57BL/6 or irrelevant CBA (H2 k ) mice that had received an intraperitoneal injection of 600 U IFN-γ 72 h earlier. The presence of GFP + Tregs in lavage, mesenteric dLNs, non-dLNs and spleen was analysed by flow cytometry 16 h later. Representative dot plots are shown in panel d . The mean number of Treg cells (in the total CD4 + population) detected in the peritoneal cavity and lymphoid organs is shown in panel e . Error bars represent s.d. Statistical significance was calculated with unpaired Student’s t -test. ( n =3, N =4) * P <0.05, ** P <0.01. Full size image Having established that antigen presentation regulates Treg recruitment, we sought to verify that recognition of endogenous peptides (putative ‘self antigens’) in the context of self-MHC class II molecules is instrumental for efficient Treg localization to target tissue. Mice expressing a transgenic TCR specific for a HY-derived peptide in the context of H2-A b (Marilyn mice) [22] were crossed with GFP-Foxp3 reporter mice and used in these experiments. The male minor histocompatibility antigen HY is encoded by the Y chromosome, is expressed by all male cells and plays a role in secondary recurrent miscarriage [23] . In male individuals, HY-specific T cells are removed in the thymus by negative selection [24] , [25] . In the F1 Marilyn GFP-Foxp3 mice, the mean percentage of CD4 + Vβ6 + Marilyn T cells as a proportion of total lymphocytes was 12.2% (±2.5%). In the same mice, the mean percentage of naturally occurring Tregs (GFP + ) as a proportion of Marilyn T cells was 3.5% (±1.4%). Purified and pooled CD4 + T cells from Marilyn GFP-Foxp3 F1 mice were injected intravenously (i.v.) in IFN-γ-treated male or female C57BL/6 syngeneic recipients (10 7 /mouse). Recipient mice are genetically identical and express the same MHC molecules, with the exception of the HY antigen, which is only expressed in male animals. The presence of GFP Foxp3 + , Vβ6 + T cells in the peritoneal lavage, dLNs and non-dLNs and the spleen was analysed by flow cytometry. As it is shown in Fig. 3a,b , Foxp3 + Vβ6 + T cells were significantly enriched in the peritoneal cavity and dLNs of male, but not female recipients. Interestingly, these experiments also revealed a redistribution of HY-specific Tregs, which were depleted from the ndLN and the spleen. 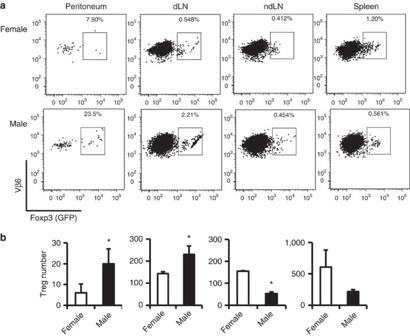Figure 3: Self-recognition drives Treg recruitment. Total CD4+T cells from GFP-Foxp3 Marilyn F1 mice (107/mouse) were injected intravenously into syngeneic male or female C57BL/6 mice that had received an intraperitoneal injection of 600 U IFN-γ 72 h earlier. An anti-Vβ6 antibody was used to identify Marilyn T cells22. The presence of GFP+Vβ6+Tregs in lavage, dLN and spleen was analysed by flow cytometry 16 h later. Tregs were identified by gating on the CD4+T-cell population. Representative dot plots are shown in panela. The mean number of Treg cells (in the total CD4+population) of Treg cells detected in the peritoneal cavity and lymphoid organs is shown in panelb. Error bars represent s.d. Statistical significance was calculated with unpaired Student’st-test. (n=3,N=2) *P<0.05. Figure 3: Self-recognition drives Treg recruitment. Total CD4 + T cells from GFP-Foxp3 Marilyn F1 mice (10 7 /mouse) were injected intravenously into syngeneic male or female C57BL/6 mice that had received an intraperitoneal injection of 600 U IFN-γ 72 h earlier. An anti-Vβ6 antibody was used to identify Marilyn T cells [22] . The presence of GFP + Vβ6 + Tregs in lavage, dLN and spleen was analysed by flow cytometry 16 h later. Tregs were identified by gating on the CD4 + T-cell population. Representative dot plots are shown in panel a . The mean number of Treg cells (in the total CD4 + population) of Treg cells detected in the peritoneal cavity and lymphoid organs is shown in panel b . Error bars represent s.d. Statistical significance was calculated with unpaired Student’s t -test. ( n =3, N =2) * P <0.05. Full size image Overall, these data suggest that recognition of endogenous peptides in the context of self-MHC class II molecules can drive Treg recruitment into non-lymphoid tissue and dLNs. IFN-γ-induced MHC class II molecules drive Treg migration The essential role of self-recognition of MHC class II:self-peptide complexes in Treg migration to target tissue was further confirmed by experiments comparing the recruitment of freshly isolated Treg from the circulation into peritoneum of IFN-γ-treated syngeneic recipients of which some received a rat anti-mouse MHC class II antibody (clone M5/114) i.v. prior to Treg transfer. As it is shown in Fig. 4a,b , masking of MHC II molecules abrogated Treg enrichment in the peritoneal cavity and dLNs. 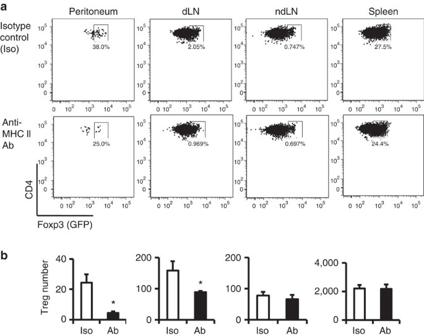Figure 4: Treg accumulation requires MHC class II molecule expression by target tissue. Total CD4+T cells isolated from FoxP3-GFP reporter mice were injected intravenously into syngeneic C57BL/6 mice (107/mouse) that had received an intraperitoneal injection of 600 U IFN-γ 72 h earlier. Prior to Treg adoptive transfer, recipient mice received either 500 μg anti-MHC class II antibody (clone M5/114, BioXCell) or isotype control antibody. The presence of GFP+Tregs in the peritoneal lavage, dLN, ndLN and spleen was analysed by flow cytometry 16 h later. Tregs were identified by gating on the CD4+GFP+population. Representative dot plots are shown in panela. The mean number of Treg cells (in the total CD4+population) detected in the peritoneal cavity and lymphoid organs is shown in panelb. Error bars represent s.d. Statistical significance was calculated with unpaired Student’st-test. (n=3,N=3) *P<0.05. Figure 4: Treg accumulation requires MHC class II molecule expression by target tissue. Total CD4 + T cells isolated from FoxP3-GFP reporter mice were injected intravenously into syngeneic C57BL/6 mice (10 7 /mouse) that had received an intraperitoneal injection of 600 U IFN-γ 72 h earlier. Prior to Treg adoptive transfer, recipient mice received either 500 μg anti-MHC class II antibody (clone M5/114, BioXCell) or isotype control antibody. The presence of GFP + Tregs in the peritoneal lavage, dLN, ndLN and spleen was analysed by flow cytometry 16 h later. Tregs were identified by gating on the CD4 + GFP + population. Representative dot plots are shown in panel a . The mean number of Treg cells (in the total CD4 + population) detected in the peritoneal cavity and lymphoid organs is shown in panel b . Error bars represent s.d. Statistical significance was calculated with unpaired Student’s t -test. ( n =3, N =3) * P <0.05. Full size image Induction of MHC class II expression is selectively induced by IFN-γ via the CIITA promoter [26] . However, IFN-γ can also induce the upregulation of adhesion molecules such as ICAM-1 ( Supplementary Fig. 2 ), which mediate lymphocyte recruitment [27] . To assess the potential contribution of other adhesion receptors to Treg recruitment to inflammatory sites, localization of GFP-tagged Tregs in the peritoneum of syngeneic recipients pre-treated with 20 ng TNFα i.p. was analysed. As shown in Fig. 5 , exposure to TNFα failed to enhance Treg recruitment ( Fig. 5a,b ) while the recruitment of endogenous monocytes within the peritoneal cavity and dLNs was increased by this cytokine ( Fig. 5c ). As TNFα does not induce MHC class II expression ( Supplementary Fig. 2 and ref. 26 ), these data further support the non-redundant role of IFN-γ in sustaining Treg trafficking to inflammatory sites. 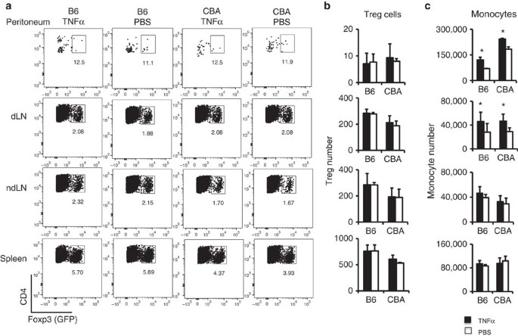Figure 5: TNF-α does not enhance the recruitment of Tregs to target tissue. Total CD4+T cells from FoxP3-GFP reporter mice (107/mouse) were injected intravenously into syngeneic C57BL/6 or irrelevant CBA mice that had received an intraperitoneal injection of 20 ng TNF-α (Peprotech) or control saline 48 h earlier. The presence of GFP+Tregs in lavage, dLN, ndLN and spleen was analysed by flow cytometry. Representative dot plots are shown in panela. The mean number of Treg cells (in the total CD4+population) present in the peritoneal lavage and lymphoid organs is shown in panelb. The recruitment of endogenous monocytes in lavage, dLN, ndLN and spleen was analysed by CD68 staining. The mean number of monocytes detected in the peritoneal cavity and lymphoid organs of at least three recipients is shown in panelc. Error bars represent s.d. Statistical significance was calculated with unpaired Student’st-test. (n=3,N=4) *P<0.05. Figure 5: TNF-α does not enhance the recruitment of Tregs to target tissue. Total CD4 + T cells from FoxP3-GFP reporter mice (10 7 /mouse) were injected intravenously into syngeneic C57BL/6 or irrelevant CBA mice that had received an intraperitoneal injection of 20 ng TNF-α (Peprotech) or control saline 48 h earlier. The presence of GFP + Tregs in lavage, dLN, ndLN and spleen was analysed by flow cytometry. Representative dot plots are shown in panel a . The mean number of Treg cells (in the total CD4 + population) present in the peritoneal lavage and lymphoid organs is shown in panel b . The recruitment of endogenous monocytes in lavage, dLN, ndLN and spleen was analysed by CD68 staining. The mean number of monocytes detected in the peritoneal cavity and lymphoid organs of at least three recipients is shown in panel c . Error bars represent s.d. Statistical significance was calculated with unpaired Student’s t -test. ( n =3, N =4) * P <0.05. Full size image The protective effect of IFN-γ signalling in models of autoimmunity has been long established, although the molecular mechanisms of this effect are at present unclear [28] . More recently, Treg function has been shown be dependent on IFN-γ [29] . We therefore sought to assess whether the requirement of this cytokine for Treg function reflects in part its ability to facilitate Treg localization to target tissue by enhancing antigen presentation. To distinguish between the impact of responsiveness to IFN-γ by either Treg cells or target tissue, experiments were performed involving either adoptive transfer of CD4 + T cells isolated by immunomagnetic negative selection from IFN-γRKO Tregs (labelled with PKH26) into wild-type (WT) syngeneic recipients, or injection of CD4 + WT T cells isolated from GFP-Foxp3 mice in IFN-γR KO syngeneic animals, in both cases following i.p. treatment with IFN-γ. As shown in Fig. 6a,b , antigen-driven recruitment of IFN-γR KO Tregs (PKH26 + , Foxp3 + ) was similar to that of WT GFP-Tregs. In contrast, inability of target tissue to respond to IFN-γ led to diminished WT Treg recruitment to the peritoneal cavity and dLN in IFN-γR KO syngeneic recipients ( Fig. 6c,d ). 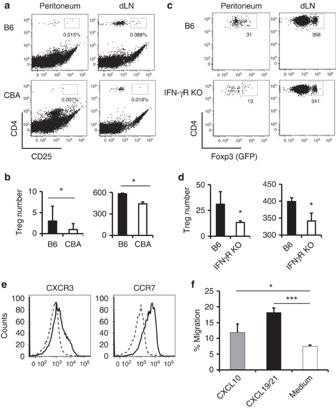Figure 6: Treg accumulation requires target tissue responsiveness to IFN-γ stimulation. (a,b) Total CD4+T cells from IFN-γ receptor KO mice (107/mouse) were labelled with 2 μM PKH26 and injected intravenously into syngeneic WT C57BL/6 or irrelevant CBA (H2k) mice that had received an intraperitoneal injection of 600 U IFN-γ 72 h earlier. The presence of PKH26+, CD4+CD25+Tregs in the peritoneal lavage and dLN was analysed by flow cytometer 16 h later. In panela, representative dot plots of IFN-γR KO Treg cells detected in the peritoneal lavage and dLN are shown. The mean number of Treg cells (in the total CD4+population) present in the peritoneal cavity and dLN is shown in panelb. Error bars represent s.d. Statistical significance was calculated with unpaired Student’st-test. (n=3,N=4) *P<0.05. (c,d) Total CD4 T cells from FoxP3-GFP reporter mice (107/mouse) were injected intravenously into WT C57BL/6 or IFN-γ receptor KO mice that had received an intraperitoneal injection of 600 U IFN-γ 72 h earlier. The presence of PKH26+, CD4+CD25+Tregs in the peritoneal lavage and dLN was analysed by flow cytometry 16 h later. Tregs were gated on CD4+GFP+population. Representative dot plots are shown in panelc. The mean number of Treg cells (in the total CD4+population) present in the peritoneal cavity and dLN is shown in paneld. Error bars represent s.d. Statistical significance was calculated with unpaired Student’st-test. (n=3,N=2) *P<0.05. The expression of CXCR3 and CCR7 by GFP+Treg cells was analysed by flow cytometry (e) and their migration in response to their respective ligands CXCL10 (300 ng ml−1) and CCL19/21 (200 ng ml−1) was assessed by a 6-h transwell assay (106/well) (f). Data are representative of three independent experiments of identical design. Error bars represent s.d. Statistical significance was calculated with unpaired Student’st-test. *P<0.05, ***P<0.001. Figure 6: Treg accumulation requires target tissue responsiveness to IFN-γ stimulation. ( a , b ) Total CD4 + T cells from IFN-γ receptor KO mice (10 7 /mouse) were labelled with 2 μM PKH26 and injected intravenously into syngeneic WT C57BL/6 or irrelevant CBA (H2 k ) mice that had received an intraperitoneal injection of 600 U IFN-γ 72 h earlier. The presence of PKH26 + , CD4 + CD25 + Tregs in the peritoneal lavage and dLN was analysed by flow cytometer 16 h later. In panel a , representative dot plots of IFN-γR KO Treg cells detected in the peritoneal lavage and dLN are shown. The mean number of Treg cells (in the total CD4 + population) present in the peritoneal cavity and dLN is shown in panel b . Error bars represent s.d. Statistical significance was calculated with unpaired Student’s t -test. ( n =3, N =4) * P <0.05. ( c , d ) Total CD4 T cells from FoxP3-GFP reporter mice (10 7 /mouse) were injected intravenously into WT C57BL/6 or IFN-γ receptor KO mice that had received an intraperitoneal injection of 600 U IFN-γ 72 h earlier. The presence of PKH26 + , CD4 + CD25 + Tregs in the peritoneal lavage and dLN was analysed by flow cytometry 16 h later. Tregs were gated on CD4 + GFP + population. Representative dot plots are shown in panel c . The mean number of Treg cells (in the total CD4 + population) present in the peritoneal cavity and dLN is shown in panel d . Error bars represent s.d. Statistical significance was calculated with unpaired Student’s t -test. ( n =3, N =2) * P <0.05. The expression of CXCR3 and CCR7 by GFP + Treg cells was analysed by flow cytometry ( e ) and their migration in response to their respective ligands CXCL10 (300 ng ml −1 ) and CCL19/21 (200 ng ml −1 ) was assessed by a 6-h transwell assay (10 6 /well) ( f ). Data are representative of three independent experiments of identical design. Error bars represent s.d. Statistical significance was calculated with unpaired Student’s t -test. * P <0.05, *** P <0.001. Full size image It has been suggested that CXCR3 is required for Treg localization to peripheral tissue [19] , [30] . As CXCR3 ligands are induced by IFN-γ, we analysed CXCR3 expression by Treg cells and their migration to its ligand CXCL10 in vitro . As it is shown in Fig. 6e,f , a relatively small fraction of Tregs expressed CXCR3 and did not migrate efficiently in response to CXCL10 compared with the CCR7 ligands CCL19 and CCL22, suggesting that lack of CXCL10 production by IFN-γRKO recipients is unlikely to significantly impact on their ability to migrate to target tissue. Altogether, these data suggest that IFN-γ facilitates Treg migration to non-lymphoid sites of inflammation and dLN by inducing expression of MHC class II molecules and self-antigen presentation by target tissue. Cognate recognition of endothelium induces Treg recruitment We and others have shown that cognate recognition of the endothelium can directly induce migration of effector T cells into non-lymphoid tissue both in vitro [31] , [32] , [33] and in vivo [34] , [35] , [36] , [37] . Recent studies reported that recruitment of Teff cell is facilitated by both endothelial cells (ECs) and perivascular DCs [38] , [39] , although DCs do not appear to directly mediate Teff migration through the endothelium [39] . Following i.p. administration of IFN-γ 72 h earlier, MHC class II molecule expression was induced in the vascular endothelium in the peritoneal membrane and dLN ( Fig. 7a and Supplementary Fig. 3 ) and was upregulated by CD11c + cells (putative DCs) in the dLN ( Supplementary Fig. 4 ). However, we failed to detect any CD11c + DCs in the peritoneal membrane ( Supplementary Fig. 5 ), and Treg migration to the dLNs of phosphate-buffered saline (PBS)-treated mice, in which DCs constitutively express MHC class II molecules ( Supplementary Fig. 4 ), was not enhanced ( Fig. 1 ). We therefore focused on the possibility that antigen display by the vascular endothelium might mediate Treg recruitment in our model. 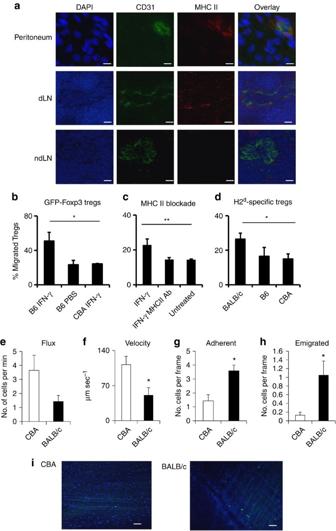Figure 7: Treg recruitment to non-lymphoid tissue is induced by cognate recognition of the vascular endothelium. (a) The peritoneal membrane, dLN and ndLNs from C57BL/6 mice that had received 600 U IFN-γ or control saline i.p. 72 h earlier were stained with anti-CD31 (green fluorescence) and anti-MHC II mAbs (red fluorescence) and analysed by wide-field fluorescence microscopy). Nuclei are highlighted by DAPI (blue). Scale bar, 10 μM. (b) Freshly isolated GFP-Tregs (106/well) were seeded onto IFN-γ or saline-treated syngeneic B6 or irrelevant CBA EC monolayers grown on transwells. The mean percentage migration measured at 6 h from three experiments of identical design is shown. *P<0.05. (c) To prevent antigen presentation, some of the IFN-γ-treated EC monolayer were exposed to an anti-MHC class II antibody (Clone M5/114, BioXcell) at 37 °C for 30 min prior to seeding the T cells. **P<0.01. (d) The mean percentage migration measured at 6 h from three experiments of identical design is shown. Error bars represent s.d. *P<0.05. (d) H2dallospecific Tregs expandedin vitro(5 × 105/well) were seeded onto IFN-γ-treated allogeneic BALB/c, syngeneic B6 and irrelevant CBA EC monolayers grown on transwells. The mean percentage migration measured at 6 h from three experiments of identical design is shown. Error bars represent s.d. **P<0.01. (e–i) Allogeneic male BALB/C and CBA/Ca (H2d, H2k) mice were treated with intrascrotal administration of IFN-γ (1,200 U in 400 μl saline). After 72 h, fluorescently labelled (CFSE) Treg cells were injected intravenously after surgical exteriorization of the cremaster muscle and T-cell interactions with venular walls were visualized and quantified by intravital microscopy for up to 40 min. (e) rolling. (f) velocity. (g) firm adhesion. (h) extravasation. Cremaster muscle sections visualized by fluorescent microscopy indicated a large tissue influx of T cells in tissues from BALB/c but not control CBA mice (i). Nuclei are stained by DAPI (blue). Results are from six mice per group, and significant differences between the H2din comparison with the H2kstrains of mice are shown by asterisk. Error bars represent s.d. *P<0.05 (N=2). Scale bar, 10 μM. In all the experiments described above statistical significance was calculated with unpaired Student’st-test. Figure 7: Treg recruitment to non-lymphoid tissue is induced by cognate recognition of the vascular endothelium. ( a ) The peritoneal membrane, dLN and ndLNs from C57BL/6 mice that had received 600 U IFN-γ or control saline i.p. 72 h earlier were stained with anti-CD31 (green fluorescence) and anti-MHC II mAbs (red fluorescence) and analysed by wide-field fluorescence microscopy). Nuclei are highlighted by DAPI (blue). Scale bar, 10 μM. ( b ) Freshly isolated GFP-Tregs (10 6 /well) were seeded onto IFN-γ or saline-treated syngeneic B6 or irrelevant CBA EC monolayers grown on transwells. The mean percentage migration measured at 6 h from three experiments of identical design is shown. * P <0.05. ( c ) To prevent antigen presentation, some of the IFN-γ-treated EC monolayer were exposed to an anti-MHC class II antibody (Clone M5/114, BioXcell) at 37 °C for 30 min prior to seeding the T cells. ** P <0.01. ( d ) The mean percentage migration measured at 6 h from three experiments of identical design is shown. Error bars represent s.d. * P <0.05. ( d ) H2 d allospecific Tregs expanded in vitro (5 × 10 5 /well) were seeded onto IFN-γ-treated allogeneic BALB/c, syngeneic B6 and irrelevant CBA EC monolayers grown on transwells. The mean percentage migration measured at 6 h from three experiments of identical design is shown. Error bars represent s.d. ** P <0.01. ( e – i ) Allogeneic male BALB/C and CBA/Ca (H2 d , H2 k ) mice were treated with intrascrotal administration of IFN-γ (1,200 U in 400 μl saline). After 72 h, fluorescently labelled (CFSE) Treg cells were injected intravenously after surgical exteriorization of the cremaster muscle and T-cell interactions with venular walls were visualized and quantified by intravital microscopy for up to 40 min. ( e ) rolling. ( f ) velocity. ( g ) firm adhesion. ( h ) extravasation. Cremaster muscle sections visualized by fluorescent microscopy indicated a large tissue influx of T cells in tissues from BALB/c but not control CBA mice ( i ). Nuclei are stained by DAPI (blue). Results are from six mice per group, and significant differences between the H2 d in comparison with the H2 k strains of mice are shown by asterisk. Error bars represent s.d. * P <0.05 ( N =2). Scale bar, 10 μM. In all the experiments described above statistical significance was calculated with unpaired Student’s t -test. Full size image This hypothesis was first assessed in vitro by measuring migration of Tregs through antigen-expressing EC monolayers. Treg were isolated from FoxP3-eGFP reporter mice [20] by cell sorting and seeded onto IFN-γ-treated syngeneic (self) EC monolayers. As a control, syngeneic untreated EC and IFN-γ-treated monolayers EC derived from irrelevant CBA/Ca mice were used. As shown in Fig. 7b , Treg migration through B6-derived EC was significantly enhanced by exposure of syngeneic EC to IFN-γ and compared with migration through IFN-γ-treated CBA/Ca EC. As expected, Treg migration through IFN-γ-treated syngeneic endothelium was reduced by pre-treating the EC monolayers with an anti-MHC class II antibody in order to prevent TCR engagement ( Fig. 7c ). Similarly, migration of B6-derived H2 d -allospecific Tregs selected by in vitro culture (see Fig. 2a–c ) through IFN-γ-treated BALB/c-derived EC monolayers was enhanced compared with that through IFN-γ-treated syngeneic C57BL/6 and irrelevant CBA-derived EC monolayers ( Fig. 7d ). Overall these in vitro experiments suggest that cognate recognition of the endothelium promotes Treg migration. To directly visualize the impact of cognate recognition of the endothelium on Treg migration into tissues, intravital microscopy was used to monitor Treg cell–EC interactions in vivo . For this purpose, events within cremasteric venules of BALB/c (H-2 d ) mice, pretreated with intrascrotal administration of IFN-γ (72 h), were quantified. CBA/Ca mice (H-2 k ) were used as a control. Similar to what we had observed in the peritoneum, no CD11c + DCs were detected in the cremaster muscle irrespectively of IFN-γ treatment ( Supplementary Fig. 5 ). Fluorescently labelled H-2 d -allospecific polyclonal Treg cells were injected intravenously, and responses within the microvascular bed viewed for up to 40 min after injection of cells. No significant differences in rolling flux were observed ( Fig. 7e ) in the different groups. However, the velocity of Treg interacting with BALB/c (H-2 d ) vessels significantly decreased and was followed by significant increases in both T-cell firm adhesion and transendothelial migration ( Fig. 7f–h and Supplementary Movies 1 and 2 ). Similar to what we observed in the in vitro studies, these results suggest that antigenic endothelium directly mediates T-cell recruitment into target tissue by specifically regulating adhesion and extravasation. In line with these results, captured in real time, dissected and sectioned cremaster muscles visualized by fluorescent microscopy indicated a large tissue influx of T cells in tissues from BALB/c but not control CBA mice ( Fig. 7i ). Antigen-driven Treg migration requires PI3K p110δ activity The observations described above prompted us to further characterize the molecular mechanism of antigen-driven Treg trafficking. PI3K p110δ activity has previously been implicated in the regulation of Treg function. Despite T cells with functionally inactive PI3K p110δ respond to IL-2 and only partially lose their ability to suppress in vitro , lack of this activity leads to a complete loss of suppressive function in vivo [40] . We have shown that Teff cells expressing a functionally inactive PI3K p110δ lose susceptibility to TCR-induced migration and fail to localize efficiently to antigenic tissue [41] . We therefore sought to investigate whether the profound defect of regulatory function of Treg with inactive p110δ selectively observed in vivo could partly be attributed to their inability to locate to antigen-rich sites. For this purpose, we used in vitro expanded Tregs with direct BALB/c allospecificity. First, we tested whether pharmacological inhibition of p110δ activity has any effect on TCR-induced migration of Tregs by an in vitro transendothelial migration assay. Tregs with direct BALB/c allospecificity were treated with the selective PI3K p110δ inhibitor IC87114 (5 μM) [41] or with PBS containing vehicle (1% dimethylsulphoxide) at 37 °C for 1 h. Migration of IC87114-treated and control-treated Tregs through IFN-γ-treated EC monolayers derived from BALB/c and irrelevant CBA mice was compared. As shown in Fig. 8a , inhibition of PI3K p110δ impaired antigen-induced migration through BALB/c-derived EC monolayers, while it did not affect the modest Tregs migration through irrelevant CBA-derived ECs. 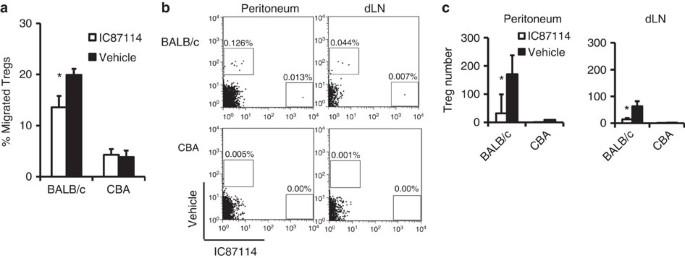Figure 8: PI3K p110δ activity is required for antigen-driven Treg recruitment. (a) H2d-allospecific Tregs were treated with 5 μM IC87114 or with vehicle control for 30 min at room temperature and subsequently washed before use. Vehicle control-treated (filled symbols) and inhibitor-treated (open symbols) T cells (5 × 105/well) were seeded onto allogeneic BALB/c and irrelevant CBA mice-derived IFN-γ-treated EC monolayers. T-cell migration measured at 6 h is shown. Data are representative of at least three independent experiments of identical design. Error bars represent s.d. Statistical significance was calculated with unpaired Student’st-test.*P<0.05. (b) BALB/c-specific Tregs were treated with 5 μM IC87114 or with vehicle control for 30 min at room temperature and subsequently washed before use. BALB/c and CBA mice were treated i.p. with 600 U IFN-γ. After 72 h, CFSE-labelled vehicle-treated Tregs and DDAO SE-labelled inhibitor-treated Tregs (107/mouse) were co-injected i.v. The presence of labelled T cells in the peritoneal cavity and dLNs was analysed after 24 h by flow cytometry. The mean number of Treg cells (in the total CD4+population) detected in the peritoneal cavity and dLNs is shown in panelc. Error bars represent s.d. Statistical significance was calculated with unpaired Student’st-test. (n=3,N=3) *P<0.05. Figure 8: PI3K p110δ activity is required for antigen-driven Treg recruitment. ( a ) H2 d -allospecific Tregs were treated with 5 μM IC87114 or with vehicle control for 30 min at room temperature and subsequently washed before use. Vehicle control-treated (filled symbols) and inhibitor-treated (open symbols) T cells (5 × 10 5 /well) were seeded onto allogeneic BALB/c and irrelevant CBA mice-derived IFN-γ-treated EC monolayers. T-cell migration measured at 6 h is shown. Data are representative of at least three independent experiments of identical design. Error bars represent s.d. Statistical significance was calculated with unpaired Student’s t -test. * P <0.05. ( b ) BALB/c-specific Tregs were treated with 5 μM IC87114 or with vehicle control for 30 min at room temperature and subsequently washed before use. BALB/c and CBA mice were treated i.p. with 600 U IFN-γ. After 72 h, CFSE-labelled vehicle-treated Tregs and DDAO SE-labelled inhibitor-treated Tregs (10 7 /mouse) were co-injected i.v. The presence of labelled T cells in the peritoneal cavity and dLNs was analysed after 24 h by flow cytometry. The mean number of Treg cells (in the total CD4 + population) detected in the peritoneal cavity and dLNs is shown in panel c . Error bars represent s.d. Statistical significance was calculated with unpaired Student’s t -test. ( n =3, N =3) * P <0.05. Full size image To confirm the requirement for p110δ activity by antigen-driven Treg migration in vivo , we compared the recruitment of IC87114- and vehicle-treated Tregs with direct BALB/c allospecificity from circulation into peritoneum of IFN-γ-treated allogeneic BALB/c and irrelevant CBA mice. DDAO SE-labelled IC87114-treated Tregs and CFSE-labelled control vehicle-treated Tregs were mixed in equal numbers and were injected i.v. into BALB/c and CBA mice that had received an i.p. injection of IFN-γ 48 h earlier. Migration of Treg cells in the peritoneal cavity and dLN was measured 16 h later. As shown in Fig. 8b,c , removal of PI3K p110δ activity significantly inhibited the recruitment of allospecific Tregs to the peritoneal cavity and dLNs of allogeneic BALB/c mice. In line with the in vitro analyses, inhibition of p110δ activity did not affect the minimal migration of Tregs into peritoneum of irrelevant CBA mice. These observations suggest that, similarly to Teff cells [41] , recruitment of Treg cells by cognate endothelium requires PI3K p110δ activation by the TCR. Tregs inhibit effector T-cell recruitment into target tissue Similarly to the initiation of effector responses, the development of regulatory mechanisms mediated by naturally occurring Treg cells is generally thought to require their initial activation in the dLNs [42] . In addition, both Treg and Teff cells rely upon similar molecular mediators (PI3K p110δ) for their recruitment by antigen-presenting endothelium [41] . Therefore, antigen-driven migration of Tregs may not be sufficient to sustain their preferential accumulation into target tissue compared with that of Teff cells. Thus, additional mechanisms must be in place, which allow the establishment of an optimal Treg:Teff ratio to terminate T-cell-mediated inflammation at the late stages of the immune response. Allospecific conventional T cells were generated by i.p. immunization of B6 mice with BALB/c splenocytes and further in vitro expansion. The allospecific T-cell population was composed of a mixture of T cells with effector (Teff) and central memory (Tcm) phenotype ( Supplementary Fig. 6 ). A comparison of allospecific (H2 d ) Treg and conventional memory T cell crawling over CBA-derived EC monolayers by time-lapse microscopy did not reveal any significant difference in their migratory speed ( Fig. 9a ). Having ruled out differences in intrinsic motility, we compared the antigen-driven migration of similar-sized populations of activated, allospecific Treg and Tcm/eff cells to target tissue. Adoptively transferred H-2 d allospecific T cells preferentially accumulated in the peritoneal cavity of IFN-γ-treated BALB/c mice ( Supplementary Fig. 7 ), as previously described [19] . However, when these T cells were co-injected with equal numbers of H-2 d allospecific Tregs, their localization to the peritoneal cavity and dLN was abrogated ( Fig. 9b,c ). In contrast, primed conventional T cells were still retrievable in the spleen and non-dLNs, suggesting that their absence in target tissue was not due to Treg-induced apoptosis [43] . These data show that once Treg cells have been recruited by antigen-presenting endothelium, they can inhibit conventional T-cell migration into the same tissue. 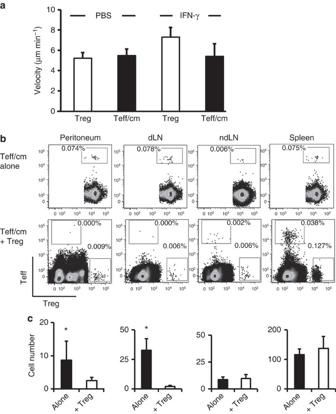Figure 9: Treg cells inhibit the recruitment of primed conventional T-cell into target tissue. (a) H2d-allospecific Treg or conventional T cells were seeded onto confluent CBA-derived EC monolayers pre-treated with IFN-γ (300 U ml−1) for 72 h. T-cell migration was monitored by timelapse microscopy. The crawling speed (μm min−1) of T cells was measured using ImageJ analysis software. About 30–40 cells were tracked in each experimental condition. Error bars represent s.d. Statistical significance was calculated with unpaired Student’st-test.N=2. (b,c) H2d-allospecific conventional T cells (107/mouse) were labelled with 1 μM DDAO SE and co-injected intravenously with CFSE-labelled H2d-allospecific Tregs (107/mouse) into BALB/C mice that had received an intraperitoneal injection of 600 U IFN-γ 72 h earlier. The presence of DDAO SE+Teff/cm and CFSE+Tregs in the peritoneal cavity, dLN, ndLN and spleen was analysed 16 h later by flow cytometry. Representative dot plots and the mean number of labelled cells present in the peritoneal lavage are shown in panelsbandc, respectively. Error bars represent s.d. Statistical significance was calculated with unpaired Student’st-test. *P<0.05 (n=3,N=2). Figure 9: Treg cells inhibit the recruitment of primed conventional T-cell into target tissue. ( a ) H2 d -allospecific Treg or conventional T cells were seeded onto confluent CBA-derived EC monolayers pre-treated with IFN-γ (300 U ml −1 ) for 72 h. T-cell migration was monitored by timelapse microscopy. The crawling speed (μm min −1 ) of T cells was measured using ImageJ analysis software. About 30–40 cells were tracked in each experimental condition. Error bars represent s.d. Statistical significance was calculated with unpaired Student’s t -test. N =2. ( b , c ) H2 d -allospecific conventional T cells (10 7 /mouse) were labelled with 1 μM DDAO SE and co-injected intravenously with CFSE-labelled H2 d -allospecific Tregs (10 7 /mouse) into BALB/C mice that had received an intraperitoneal injection of 600 U IFN-γ 72 h earlier. The presence of DDAO SE + Teff/cm and CFSE + Tregs in the peritoneal cavity, dLN, ndLN and spleen was analysed 16 h later by flow cytometry. Representative dot plots and the mean number of labelled cells present in the peritoneal lavage are shown in panels b and c , respectively. Error bars represent s.d. Statistical significance was calculated with unpaired Student’s t -test. * P <0.05 ( n =3, N =2). Full size image The reciprocal dynamics of effector T lymphocytes and naturally occurring CD4 + CD25 + Foxp3 + Treg cells localization to lymphoid and non-lymphoid tissue are instrumental to an efficient yet regulated immune responses. Treg homing to dLNs and non-lymphoid target tissue are required for their function [5] , [6] , [7] . Remarkably, regulation of effector responses involves accumulation of a minute population of circulating Tregs into the tissue to reach an optimal Treg:Teff ratio [11] . In this study, we show that Treg trafficking is facilitated by self-recognition of MHC II: peptide complexes displayed by the endothelium of target tissue and dLNs. In turn Tregs inhibit the recruitment of activated Teff cells to the same site, thus favouring the establishment of optimal Treg:Teff ratios. This concept is well illustrated by studies investigating Treg function in allotransplantation. The frequency of directly alloreactive Tregs has been estimated to be over 10% [44] . Despite this high frequency, MHC-mismatched vascularized tissue grafts are rejected acutely via direct allorecognition [45] . The possibility that this cohort of allospecific Tregs is not numerically sufficient to prevent rejection relative to the high frequency of allospecific conventional T cells does not fully explain the lack of regulation of alloresponses. In fact, even the adoptive transfer of large numbers of polyclonal Tregs is relatively inefficient at inhibiting acute rejection compared with the delivery of Tregs with selected specificity for the alloantigen [10] , [45] . Based on the observations described here, the absence of cognate endothelium in the graft might be the main cause of the inefficient Treg-mediated regulation of alloresponses. Given that Tregs are self-specific, most Tregs would promptly recognize self-MHC:peptide complexes on autologous endothelium and migrate into target tissue to suppress, for instance, autoimmune responses. In transplantation, only a fraction of recipient Tregs would cross-react to allogeneic endothelium and gain access to the allograft in sufficient numbers to regulate the alloresponse. In addition, unlike conventional T-cell activation, which is topographically restricted to the LNs, Treg cells can also be activated in non-lymphoid target tissue itself, and subsequently migrate to the draining lymphoid stations [46] . In the absence of cognate endothelium, the delayed and inefficient recruitment of Tregs in allografts might also result in their impaired activation. In line with this hypothesis, a recent study analysing the dynamics of alloimmune response in vivo demonstrated rapid invasion of effector cells in the grafts followed by delayed arrival of Tregs that were ineffective at controlling tissue damage [11] . Similarly, in therapeutic settings, allospecific Tregs are far superior to autologous Tregs in preventing graft rejection [10] , [45] . These observations also support the notion that the regulatory response is kick-started by the release of IFN-γ and subsequent induction of MHC class II molecule expression by the endothelium of target tissue. Given that naturally occurring CD4 + CD25 + Foxp3 + Tregs produce little or no IFN-γ upon activation [47] , their mobilization would require the production of this cytokine by other sources, such as activated T cells. Hence, the strict dependence of Treg recruitment on IFN-γ might allow the coordination of sequential migratory events by Teff and Treg cells during a physiologic immune response, and ultimately orchestrate the synchronized development of effector and regulatory activities. As modelled in Fig. 10 , local upregulation of MHC class II molecules induced by IFN-γ produced by primed conventional T cells might enhance the recruitment and activation of Tregs in the dLN, and the subsequent inhibition of conventional T-cell expansion. A similar sequence of events might occur following the migration of Teff cells to target tissue. Here, IFN-γ-secreting Teff cells would support the subsequent entry of Tregs and the dampening of T-cell-mediated inflammation. In a negative feedback loop, Treg access to target tissue could in turn prevent the further entrance of Teff cells, leading to the resolution of inflammation. 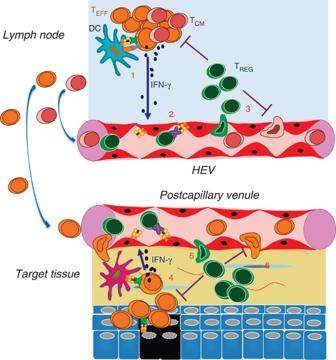Figure 10: IFN-γ-induced MHC expression by the endothelium coordinates effector and regulatory responses in lymphoid and non-lymphoid tissue. Naïve T cells are activated in the LN, differentiate into T effector (Teff) and T central memory (Tcm) and produce IFN-γ (1). IFN-γ induces the expression of MHC class II: autologous peptide complexes by the endothelium, which are recognized by Tregs (2). This event enhances the recruitment of Tregs into the LN, where they are themselves activated and subsequently inhibit T-cell expansion, differentiation and recruitment of Tcm cells (3). Teff cells migrate to the antigen-rich peripheral tissue, where they are re-activated and produce IFN-γ (4). As a consequence of the induction of MHC class II: autologous peptide complexes expression by the endothelium, Treg cells are recruited to non-lymphoid target tissue (5). Once in the tissue, Tregs inhibit effector responses (tissue damage, indicated by the dying grey cells) and further recruitment of Teff into the tissue (6). Figure 10: IFN- γ -induced MHC expression by the endothelium coordinates effector and regulatory responses in lymphoid and non-lymphoid tissue. Naïve T cells are activated in the LN, differentiate into T effector (Teff) and T central memory (Tcm) and produce IFN-γ (1). IFN-γ induces the expression of MHC class II: autologous peptide complexes by the endothelium, which are recognized by Tregs (2). This event enhances the recruitment of Tregs into the LN, where they are themselves activated and subsequently inhibit T-cell expansion, differentiation and recruitment of Tcm cells (3). Teff cells migrate to the antigen-rich peripheral tissue, where they are re-activated and produce IFN-γ (4). As a consequence of the induction of MHC class II: autologous peptide complexes expression by the endothelium, Treg cells are recruited to non-lymphoid target tissue (5). Once in the tissue, Tregs inhibit effector responses (tissue damage, indicated by the dying grey cells) and further recruitment of Teff into the tissue (6). Full size image This scenario is also indirectly supported by our observation that the simultaneous targeting of Treg and Teff/cm cells to antigen-rich tissue totally abrogates Teff/cm cell access to the tissue. Hence, the concomitant arrival of Treg and Teff/cm to target tissue would preclude the occurrence of an effector response. In contrast, both populations co-localized in non-dLN and spleen of IFN-γ-treated recipients, suggesting that Treg cells must be activated as a consequence of local IFN-γ production (by conventional T-cells) for this effect to occur. The mechanism(s) by which Tregs prevent primed conventional T-cell access to target tissue is at present unclear. Given that migrating Tregs are first engaged by cognate endothelium in our model, it is possible that they modulate molecular interactions involved in the extravasation cascade. We have previously reported that anergic Treg cells can inhibit recruitment of Teff cells to target tissue in vivo by inactivating locally produced chemokines via dipeptidyl peptidase activity [48] . Similarly, Tregs have been shown to suppress chemokine production in dLNs, thus favouring the release of Teff at the early stages of immunity against viral infections [49] . In addition, Treg cells can prevent stable conjugate formation between DC and Teff cells in the LN in vivo [50] , [51] , although the mechanism underlying this property is unclear. Treg can also modulate T-cell exit from dLNs by indirect mechanisms including the inhibition of cytokine production and expression of chemokine receptor by conventional T cells [52] , and prevent the migration of DCs from islet allografts to the dLN in a TGFβ and IL-10-dependent fashion [46] . Further studies are needed to identify the molecular mechanism/s of this relatively novel function of Tregs, which we propose to be instrumental to the establishment of Treg:Teff ratios optimal for cell-mediated immunoregulation. Mice All mice used in this study were between the ages of 7–11 weeks. Male C57BL/6, BALB/c and CBA/ca mice were purchased from Charles River (UK) and IFN-γR KO mice were purchased from The Jackson Laboratory (USA). Foxp3/GFP knock-in female mice on the C57BL/6 background were kindly provided by Dr B Malissen (Centre d’Immunologie de Marseille-Luminy, Marseille, France). Marilyn female mice, bearing a transgenic TCR specific for the male minor transplantation antigen HY peptide epitope NAGFNSNRANSSRSS and restricted by H2-A b , have been previously described [22] . These mice were bred on a recombination activating gene 2 deficient (RAG2 −/− ) background. All the in vivo experiments were conducted under the Home Office regulation following approval by the Queen Mary Unversity of London Ethics Committee. Reagents The PI3K p110δ-selective inhibitor IC87114 was purchased from Stratech. IC87114 inhibits p110δ kinase activity in cells with an IC50 between 0.1 and 0.5 μM, and only shows cross-reactivity with other PI3K isoforms at concentrations above 10 μM [53] , [54] . We have previously shown that, at the dose used in this study (10 μM), IC87114 i does not affect the p110gamma/DOCK2/AKT pathway, which mediate T-cell responses to chemokines [41] . The cell linker PKH26 was purchased from Sigma-Aldrich and used at 2 μM. Fluorescent dye DDAO SE and CFSE were purchased from Invitrogen and used at 1.5 and 20 μM, respectively. The cytokines TNF-α and IFN-γ and the chemokines CXCL10, CCL19 and CCL21 were purchased from PeproTech EC Ltd. Blocking anti-mouse MHC Class II antibody was purchased from BioXCell. Antibodies and flow cytometry For immunohistochemistry, the following antibodies were used: rabbit polyclonal anti-mouse CD31 (1:50) was from Abcam; Armenian hamster purified anti-mouse CD11c (1:50), purified rat anti-mouse CD31 (1:50) and rat purified anti-mouse MHC Class II (I-A/I-E, clone M5/114.15.2, 1:100) were from Biolegend; Alexa Fluor 555-conjugated Goat Anti-Rat IgG (H+L) (1:100), Alexa Fluor 488-conjugated donkey Anti-Rabbit IgG (H+L) and Alexa Fluor 488-conjugated Goat Anti-Hamster IgG (H+L) (1:100) were purchased from Invitrogen/Life Technologies. All flow cytometry antibodies were used at 1:100 dilutions unless otherwise specified. Purified rat anti-mouse MHC Class II (I-A/I-E, clone M5/114.15.2), FITC-conjugated anti-mouse CD54 (ICAM-1, clone YN1/1.7.4), PE-conjugated anti-mouse CD86 (B7-2, clone GL-1) were purchased from Biolegend; PE-conjugated anti-mouse CD80 (B7-1, clone 3H5), FITC-conjugated anti-mouse CD106 (VCAM-1, clone 429), PE-Cy7-conjugated anti-mouse CD25 (clone PC61.5), PE-conjugated anti-mouse CXCR-3 (clone CXCR3-173), PE-conjugated anti-mouse CCR7 (clone 4B12), PE-conjugated anti-mouse CCR4 (clone 2G12), PE-conjugated anti-mouse CCR5 (clone HM-CCR5(7A4)), PE-conjugated anti-mouse CD11a (LFA-1,clone M17/4) PE-conjugated anti-mouse CD31 (PECAM-1, clone 390), PE-conjugated anti-mouse CD62L ( L -Selectin, clone MEL-14), efluor 450-conjugated anti-mouse CD44 (clone IM7), PE-Cy7-conjugated anti-mouse CD69 (clone H1.2F3), PE-conjugated anti-mouse CXCR4 (clone 2B11), PE-conjugated anti-mouse α4 β7 (clone DATK32), FITC-conjugated anti-mouse CD8 (clone 53-6.7) and APC-conjugated anti-FOXP3 (clone FJK-16s) were purchased from eBioscience; PE Texas red-conjugated anti-mouse CD4 (clone RM4-5) and Alexa fluor 488-conjugated Goat anti-Rat Antibody (1:200) were purchased from Invitrogen. For intracellular Foxp3 staining, the Anti-Mouse/Rat Foxp3 Staining Set APC from eBioscience was used according to manufacturer’s instructions. For surface staining, cells were labelled with the appropriate concentration of fluorescence-conjugated antibodies or isotype control according to manufacturer’s instructions, and analysed by a four-laser BD LSRFortessa (BD Biosciences). Acquired samples were analysed using Flowjo 7.6 (TreeStar Inc.). Lymphocyte transmigration assays Murine vascular ECs were isolated from mouse lungs [55] . ECs were treated with 600 U ml −1 IFN-γ (PeproTech, London, UK) for 48–72 h to induce upregulation of Class II MHC molecules. A total of 3 × 10 4 IFN-γ treated ECs were seeded and cultured on gelatin-coated (Sigma) Transwell tissue culture well inserts (diameter, 6.5 mm) containing 3-μm pore size (Costar) polycarbonate membranes for 16 h to from a monolayer. T cells (5 × 10 5 ) in RPMI 1640 supplemented with 2% fetal bovine serum (Sera laboratories International Ltd) were added into each insert and left to migrate through the monolayer; the well volume was also replaced with fresh media. The number of migrated T cells was determined by hemocytometric counting of the cells present in the well media at different time points over a 24-h period. Results are expressed as percentage of transmigrated cells. Lymphocyte chemokinesis assays About 5–10 × 10 5 T cells were seeded onto Transwell tissue culture well inserts (diameter, 6.5 mm) with 5-μm pore size (Costar, High Wycombe, UK) polycarbonate membranes and chemokine containing media was placed in the bottom of the well. The number of migrated cells was determined by hemocytometric counting of the cells present in the well media at indicated time points. Results are expressed as percentage of transmigrated cells. Generation of H2 d -allospecific Treg cells CD4 + CD25 + Treg cells were isolated from spleen and LNs using the EasySep immunomagnetic isolation kit (StemCell Technologies SARL). To expand H2 d -allospecific CD4 + CD25 + Tregs, cells isolated from C57BL/6 mice were stimulated weekly with irradiated immature BALB/c-derived DCs at a ratio of 5:1 (Treg:DC). The co-cultures were maintained in RPMI 1640 supplemented with 10% heat inactivated foetal bovine serum (Sera laboratories International Ltd), 2 mM glutamine (Gibco), 100 U ml −1 penicillin (Gibco), 100 μg ml −1 streptomycin (Gibco), 1 mM sodium pyruvate (Gibco), 10 mM HEPES (Gibco), 50 μM 2-mercaptoethanol (Gibco) and 10 U ml −1 IL-2 in a 24-well plate. Cells were harvested and seeded at an optimal density of 1.5 × 10 6 Treg cells per well of the 24-well plate each week. Timelapse microscopy About 5–7 × 10 4 murine ECs were seeded onto wells of a 24-well tissue culture plate to obtain confluent monolayers. A total of 5 × 10 5 Treg or Teff/cm cells were seeded onto confluent endothelial monolayers and their migration was recorded using a Nikon Eclipse TE2000 microscope, equipped with a × 20 objective and Metamorph software (Molecular Devices LLC). Images were taken every minute for a 60-min period and the migration speed (μm min −1 ) of the cells was determined using ImageJ analysis software. About 30–40 cells were tracked in each experimental condition. Intravital microscopy T cell–EC interactions were visualized by intravital microscopy of the cremasteric muscle vasculature of male mice pre-treated with intrascrotal injection of 1,200 U IFN-γ for 72 h. Mice were then anesthetized by IP administration of ketamine (150 mg kg −1 ) (Ketalar; Parke-Davis, Cambridge, UK) and 7.5 mg kg −1 xylazine (Rompun; Bayer, Newbury, UK) and placed on a custom-built, heated (37 °C) microscope stage. The jugular vein was cannulated and the cremaster muscle was exteriorized through an incision in the scrotum. One testis was gently drawn out to allow the cremaster muscle to be opened and pinned outflat over the optical window within the microscope stage. The tissue was kept warm and moist throughout each experiment by superfusion with 37 °C bicarbonate buffered saline. A total of 2.5 × 10 7 CFSE (20 μm) labelled T cells were infused into the cannulated jugular vein and the cremaster muscle post capillary venules were imaged 1 h later using an Olympus BX61W1 microscope with an Olympus UMPlanFL × 20/0.50 W water immersion objective (Carl Zeiss Ltd.). The set-up was connected to an Olympus BXUCB lamp, Uniblitz VCMD1 shutter driver and DG4-700 shutter instrument. The set-up used a Hamamatsu C9300 digital camera with a Videoscope VS4-1845 image intensifier attached. All videos were captured and analysis carried out using Slidebook 5.0 software (Intelligent Imaging TTL). Rolling cells were defined as fluorescent T cells moving slower than the flowing erythrocytes, and rolling flux was quantified as the number of rolling cells moving past a fixed point on the venular wall per 5 min. Firmly adherent leukocytes were defined as fluorescent T cells that remained stationary for at least 30 s within a 450 um vessel segment. Transmigrated cells were defined as those cells in the extravascular tissue of the 340–450 μm field of view, either side of the vessel segments quantified. at least two sections of 2–5 vessels were studied in each animal. Widefield fluorescence microscopy Tissues were sampled and embedded in Optimal Cutting Temperature compound (OCT; Agar Scientific), snap-frozen and stored until analysis. Frozen tissue sections were laid onto Polysine Microscope slides (VWR International), air dried and then fixed with ice cold acetone for 10 min. Tissue sections were washed in PBS, blocked with PBS containing 2% goat and rabbit serum and stained using rabbit anti-mouse CD31 (Abcam), rat anti-mouse MHCII antibodies (BioXCell) antibodies at 4 °C for 24 h. Excess antibody was washed away with PBS and tissues were stained with indicated secondary antibodies along with DAPI (4',6-diamidino-2-phenylindole) (Invitrogen/Life Technologies) for 30 min at room temperature. Slides were washed, mounted in ProLong Gold Antifade Reagent (Invitrogen/Life Technologies, Paisley, UK) and visualized using a Zeiss Z1 fluorescence microscope (Carl Zeiss, Cambridge, UK) equipped with an AxioCam MRm Cooled monochrome digital camera and an Apotome 2 Imaging unit. Images were acquired using a Plan Apochromat 20x/0.8 NA objective and Axiovision software version 4.8. Statistical analysis Results are expressed as mean standard error of the mean (s.e.m.) or mean s.d. To assess significance, unpaired Student’s t -tests were performed. A P -value of <0.05 was regarded as significant. How to cite this article: Fu, H. et al. Self-recognition of the endothelium enables regulatory T-cell trafficking and defines the kinetics of immune regulation. Nat. Commun. 5:3436 doi: 10.1038/ncomms4436 (2014).